Large-scale single-chirality separation of single-wall carbon nanotubes by simple gel chromatography Monostructured single-wall carbon nanotubes (SWCNTs) are important in both scientific research and electronic and biomedical applications; however, the bulk separation of SWCNTs into populations of single-chirality nanotubes remains challenging. Here we report a simple and effective method for the large-scale chirality separation of SWCNTs using a single-surfactant multicolumn gel chromatography method utilizing one surfactant and a series of vertically connected gel columns. This method is based on the structure-dependent interaction strength of SWCNTs with an allyl dextran-based gel. Overloading an SWCNT dispersion on the top column results in the adsorption sites of the column becoming fully occupied by the nanotubes that exhibit the strongest interaction with the gel. The unbound nanotubes flow through to the next column, and the nanotubes with the second strongest interaction with the gel are adsorbed in this stage. In this manner, 13 different ( n , m ) species were separated. Metallic SWCNTs were finally collected as unbound nanotubes because they exhibited the lowest interaction with the gel. Conceptually, a single-wall carbon nanotube (SWCNT) is a hollow cylinder formed by rolling up a graphene sheet [1] . The direction and magnitude of the rolling vector define the chiral angle and diameter, respectively, of the resulting nanotube. These geometric parameters determine the electrical properties of the nanotube [1] . For example, SWCNTs can be either metallic (M) or semiconducting (S) depending on their chiral angles and diameters [1] . Moreover, the energy bandgap of S-SWCNTs is inversely proportional to the nanotube diameter [2] , [3] . However, many advanced applications of SWCNTs (such as conductive films [4] , [5] , high-performance field-effect transistors [6] , nanoscale sensors [7] and optical devices [8] ) require a population of nanotubes with well-defined structures and electrical properties. The current processes for SWCNT growth generally produce complex mixtures that contain many chiralities. Consequently, there have been intense efforts to develop various postgrowth techniques for separating SWCNTs, including selective chemistry [9] , [10] , dielectrophoresis [11] , selective oxidation [12] , electrical breakdown [13] , ultracentrifugation [14] , [15] , [16] and DNA wrapping chromatography [17] , [18] , [19] , [20] . Several of these methods have been demonstrated to achieve high-purity separation of M- and S-SWCNTs. DNA wrapping and ultracentrifugation can even be used to separate nanotubes to single chirality. However, these powerful nanotube separation methods suffer from problems such as low yields and high cost. Our group recently developed a technique that uses agarose gel chromatography to separate M- and S-SWCNTs at a large scale [21] , [22] , [23] , [24] . We observed that using agarose gel as the medium for gel column chromatography required the use of a surfactant solution with a high dispersibility (such as sodium deoxycholate) to elute the bound S-SWCNTs. Successively increasing the sodium deoxycholate concentration during collection of S-SWCNTs permitted low-resolution diameter separation [24] , but further chirality separation was not possible. These results indicate that agarose gel interacts strongly with S-SWCNTs of various structures, but it has a low selectivity. Moshammer et al . [25] successfully separated M- and S-SWCNTs using an allyl dextran-based size-exclusion gel (Sephacryl S-200, GE Healthcare). In this study, we used this gel as the medium and devised a single-surfactant multicolumn gel chromatography (SS-MUGEC) method, in which several gel columns are connected vertically in series to achieve large-scale chirality separation. Loading an excess amount (that is, overloading) of SWCNT dispersion in a sodium dodecyl sulphate (SDS) aqueous solution onto the top column resulted in the selective adsorption of S-SWCNTs with different chiralities in the various columns on the basis of the strengths of their interactions with the gel. Metallic nanotubes exhibited the lowest interaction with the gel and so were finally collected as unbound nanotubes. By performing a second separation of each S-SWCNT fraction to improve chirality purity level, we successfully isolated 13 major ( n , m ) species from a high-pressure carbon monoxide (HiPco)-grown mixture [26] . Overloading effect To investigate the overloading effect, we prepared two columns (Cols. 1 and 2), each filled with the same amount (1.4 ml) of allyl dextran-based size-exclusion gel ( Fig. 1a ). A total of 1- and 8-ml SWCNT dispersions in a 2 wt% aqueous SDS solution were applied to Cols. 1 and 2, respectively. After elution of the unbound nanotubes with a low-concentration (2 wt%) SDS aqueous solution, the colours of the two columns were different ( Fig. 1b ). The top of Col. 1 was purple, and it became increasingly blue down the column, whereas Col. 2 was a uniform purple. After injecting a high-concentration (5 wt%) SDS solution, the S-SWCNT solution collected from Col. 1 was a deep blue, whereas that from Col. 2 was purple ( Fig. 1c ). This colour difference clearly demonstrates that nanotubes with different structures were selectively adsorbed by the two gel columns. A video of the separation process illustrates this result (see Supplementary Movie 1 ). 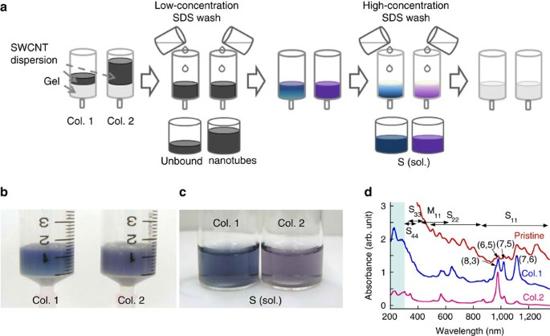Figure 1: Effect of overloading single-wall carbon nanotubes (SWCNTs) on gel columns. (a) Schematic diagram of overloading effect with SWCNTs in the gel columns. One- and 8-ml aliquots of SWCNT dispersion were loaded into Col. 1 and Col. 2, respectively. (b) Photograph of the gel columns after washing the unbound nanotubes. (c) Photograph of the collected S-SWCNT solutions from Cols. 1 (left) and 2 (right). (d) Optical absorption spectra of nanotubes selectively adsorbed in the gel columns. The spectrum for the HiPco (pristine) SWCNTs was measured as a reference. The blue shaded region (200–300 nm) indindicates the ultraviolet optical absorption characteristic of the nanotubes. (Col., column; S, semiconducting; sol., solution). Figure 1: Effect of overloading single-wall carbon nanotubes (SWCNTs) on gel columns. ( a ) Schematic diagram of overloading effect with SWCNTs in the gel columns. One- and 8-ml aliquots of SWCNT dispersion were loaded into Col. 1 and Col. 2, respectively. ( b ) Photograph of the gel columns after washing the unbound nanotubes. ( c ) Photograph of the collected S-SWCNT solutions from Cols. 1 (left) and 2 (right). ( d ) Optical absorption spectra of nanotubes selectively adsorbed in the gel columns. The spectrum for the HiPco (pristine) SWCNTs was measured as a reference. The blue shaded region (200–300 nm) in d indicates the ultraviolet optical absorption characteristic of the nanotubes. (Col., column; S, semiconducting; sol., solution). Full size image To determine the compositions of the nanotubes adsorbed from the 1- and 8-ml aliquots of the SWCNT dispersion, we measured the optical absorption spectra using an ultraviolet-visible-near-infrared spectrophotometer (Shimadzu, UV-3700). The optical absorption spectra ( Fig. 1d ) confirm that the nanotubes adsorbed in each column were enriched with S-SWCNTs but had different diameter distributions. For the 1-ml SWCNT dispersion, the adsorbed nanotubes included several chiralities and a wide diameter distribution. For the 8-ml SWCNT dispersion, the adsorbed nanotubes exhibited a much narrower diameter distribution and were highly enriched with (6, 5) nanotubes (also see Supplementary Fig. S1 ). These results demonstrate that increasing the amount of SWCNT dispersion loaded (that is, overloading) enhances the selective adsorption of S-SWCNTs with a specific chirality in a gel column. The selective adsorption of S-SWCNTs in a gel column suggests that nanotubes with different structures undergo different interactions with the gel. A particular gel column has specific effective adsorption sites. Nanotubes with the strongest interaction with the gel are adsorbed first and occupy the adsorption sites in the gel column. The other nanotubes are then adsorbed and occupy the remaining adsorption sites. As the loading amount of SWCNT dispersion is increased, the nanotubes exhibiting the strongest interaction with the gel eventually replace the other nanotubes and occupy all the adsorption sites. In this manner, a population of nanotubes with an identical structure is produced. Chirality separation by multicolumn gel chromatography The selective adsorption of S-SWCNTs on an allyl dextran-based gel column suggests that S-SWCNTs can be gradually and selectively separated by diameter based on the magnitude of their interaction strength with the gel by repeatedly loading unbound nanotubes onto a gel column. However, this is a tedious and inefficient iterative process for completely separating S-SWCNTs from M-SWCNTs. To simplify this process, we proposed the SS-MUGEC method, in which several gel columns are connected vertically in series ( Fig. 2a ). An SWCNT dispersion is applied to the top column. As the amount of the SWCNT dispersion loaded is increased, the nanotubes with the strongest interaction with the gel gradually replace other nanotubes and occupy all the adsorption sites in the top column, and the unbound nanotubes flow into the second column. The same process occurs in the second column;that is, among the unbound nanotubes, the nanotubes with the strongest interaction with the gel replace the other nanotubes and eventually occupy all the adsorption sites in the second column. Finally, nanotubes with different structures are sorted across the different columns on the basis of the strength of their interaction with the gel. Because they exhibit the lowest level of interaction with the gel, the metallic nanotubes are finally collected as unbound nanotubes. The S-SWCNTs in each column are collected by elution with high-concentration (5 wt%) aqueous SDS solution ( Supplementary Fig. S2 ). 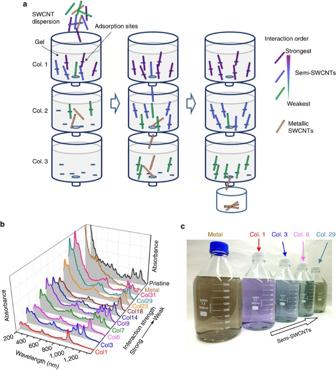Figure 2: Chirality separation of SWCNTs using single-surfactant multicolumn gel chromatography (SS-MUGEC). (a) Schematic diagram of SS-MUGEC for separating SWCNTs. (b) Optical absorption spectra and (c) photograph of the separated metallic and semiconducting SWCNT fractions (2,000 ml per fraction, ~0.8 μg ml−1). Inb, the relative interaction strength between SWCNTs and the gel is indicated with an arrow (Col., column; Semi, semiconducting). Figure 2: Chirality separation of SWCNTs using single-surfactant multicolumn gel chromatography (SS-MUGEC). ( a ) Schematic diagram of SS-MUGEC for separating SWCNTs. ( b ) Optical absorption spectra and ( c ) photograph of the separated metallic and semiconducting SWCNT fractions (2,000 ml per fraction, ~0.8 μg ml −1 ). In b , the relative interaction strength between SWCNTs and the gel is indicated with an arrow (Col., column; Semi, semiconducting). Full size image Figure 2b shows the optical absorption spectra of the nanotubes collected from the various columns and that of the unbound metallic nanotubes, with the spectrum of pristine HiPco SWCNTs provided as a reference. These absorption spectra confirm that the nanotubes bound in each gel column were highly enriched with semiconductor nanotubes, whereas the unbound nanotubes were highly enriched with metallic nanotubes. Moreover, for the S-SWCNT fractions from the first to the last column, the E 11 optical absorbance peaks in the range of 850−1,350 nm shift towards longer wavelengths, indicating that the nanotubes with smaller diameters interacted more strongly with the gel and were initially adsorbed on the gel column; this effect resulted in the separation of S-SWCNTs based on their diameter and bandgap. Figure 2b also indicates that the optical absorbance intensity of the separated nanotubes in the ultraviolet (UV) region (200−300 nm) greatly increased with increasing nanotube diameter. Recently, the dependence of nanotube UV absorbance wavelength on tube diameter has been experimentally demonstrated [27] , but the variation of absorbance intensity with tube diameter was not observed. Here the successful observation of a strong correlation between the extinction coefficient in the UV region and tube diameter is possibly due to the narrow diameter distribution of the separated nanotubes. Chirality separation of S-SWCNTs by the SS-MUGEC method was further confirmed by both the Raman spectra ( Supplementary Fig. S3 ) and photoluminescence (PL) contour maps (see Supplementary Fig. S4 ) of the S-SWCNT fractions. The various S-SWCNT fractions exhibited significant differences in their diameter and chirality distributions. More importantly, our proposed SS-MUGEC method is highly efficient and high yielding. When each column was filled with 1.4 ml of gel beads, ~24 μg of separated nanotubes were produced from each gel column. In this study, each series of columns usually contained six columns. In practice, 10 series of six columns (60 columns) can be operated concurrently because of the simplicity of the separation process; thus, ~1.44 mg of separated nanotubes can be generated in a single run. Using this method, we easily produced ~50 mg of separated nanotubes in 36 repetitions of separation runs. Figure 2c shows a photograph for 2,000 ml (~0.8 μg ml −1 ) each of solutions of the separated metallic and semiconducting nanotubes with different diameters. Single-chirality separation Figure 2 shows that, after the first separation of HiPco SWCNTs by the SS-MUGEC method, both M/S separation and chirality separation of nanotubes were achieved. However, each S-SWCNT fraction still contained several chiralities. Further separation of these S-SWCNTs fractions to achieve nanotube fractions with single chirality is highly desirable. Because the SS-MUGEC method uses the same surfactant (that is, a high-concentration SDS aqueous solution) to collect the S-SWCNTs, repeated separation of each S-SWCNT fraction can be easily performed after a simple dilution of the SDS solution [28] . 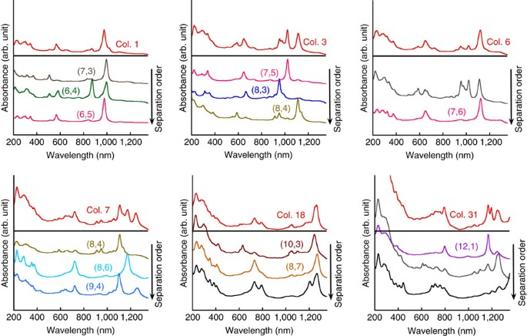Figure 3: Optical absorption spectra of nanotube fractions sorted in the second separation. In each spectral pattern, the top spectrum corresponds to one of the first separated S-SWCNT fractions, and the lower spectra are the optical absorbances of the corresponding second separated S-SWCNT fractions. The arrows indicate the separation order of the S-SWCNT fractions in the second separation (Col., column; S, semiconducting). Figure 3 shows the optical absorption spectra of the S-SWCNT fractions obtained after the second separation. The top spectra represent the optical absorbances of the S-SWCNT fractions after the first separation, whereas the lower spectra show the optical absorbances of the corresponding S-SWCNT fractions after the second separation. The separation order is indicated by an arrow. The spectra clearly indicate that each S-SWCNT fraction was further separated. After the second separation, some of the S-SWCNT fractions exhibited a main or single S 11 , S 22 , S 33 or S 44 peak [2] , suggesting that high-purity fractions containing S-SWCNTs with a single chirality were obtained. On combining the first and second chirality separation orders of S-SWCNTs, we concluded that the general separation index of single-chirality nanotubes from a HiPco mixture is as follows: (7, 3), (6, 4), (6, 5), (7, 5), (8, 3), (8, 4), (7, 6), (8, 6), (9, 4), (10, 2), (10, 3), (8, 7) and (12, 1). 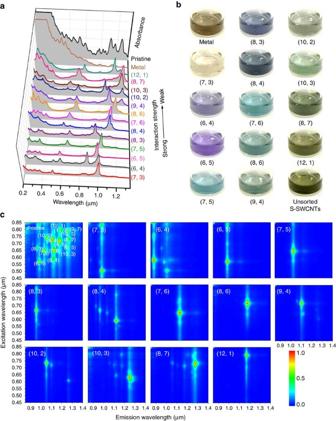Figure 4: Separated single-chirality and metallic SWCNTs. (a) Optical absorption spectra of 13 (n,m) semiconducting species together with those of metallic and pristine HiPco mixtures. The spectra are ranked according to interaction strength between the (n,m) species and the gel (that is, their separation order), as indicated by the arrow. (b) Photographs of various (n,m) species, showing their distinct colours. (c) Photoluminescence contour maps of separated (n,m) fractions. Each fraction is highly enriched with a single semiconducting species. The optical absorption spectra of these single-chirality species are compiled in Figure 4a on the basis of their separation order (that is, the interaction strength between ( n , m ) and the gel). This figure clearly indicates that 13 major single-chirality species were isolated from HiPco nanotubes after two separations. S 11 , S 22 , S 33 and S 44 peaks are clearly visible for each single-chirality S-SWCNT fraction ( Supplementary Fig. S5 ). In addition, the wavelength and intensity of the UV optical absorbance (200–300 nm) varied among the various ( n , m ) fractions. An increase in the UV absorbance wavelength and intensity of S-SWCNT fractions was observed to follow the separation order. Recently, Takagi and Okada [29] theoretically demonstrated that the absorption spectrum in the UV region depended strongly not only on nanotube diameter but also on the chiral index. They suggested that these UV spectral features are characteristic of the interband transitions near the M point of the hexagonal Brillouin zone of graphene. This structure-dependent UV optical absorption feature should be useful for further investigations of the electronic and optical properties of single-chirality species. Figure 4b presents photographs of solutions of the separated metallic nanotubes and ( n , m ) nanotubes. The distinct difference in the colours of these nanotube solutions further demonstrates the successful separation of single-chirality nanotube populations. Figure 3: Optical absorption spectra of nanotube fractions sorted in the second separation. In each spectral pattern, the top spectrum corresponds to one of the first separated S-SWCNT fractions, and the lower spectra are the optical absorbances of the corresponding second separated S-SWCNT fractions. The arrows indicate the separation order of the S-SWCNT fractions in the second separation (Col., column; S, semiconducting). Full size image Figure 4: Separated single-chirality and metallic SWCNTs. ( a ) Optical absorption spectra of 13 ( n , m ) semiconducting species together with those of metallic and pristine HiPco mixtures. The spectra are ranked according to interaction strength between the ( n , m ) species and the gel (that is, their separation order), as indicated by the arrow. ( b ) Photographs of various ( n , m ) species, showing their distinct colours. ( c ) Photoluminescence contour maps of separated ( n , m ) fractions. Each fraction is highly enriched with a single semiconducting species. Full size image The purity of single-chirality nanotubes is important in electronic applications. In this study, the main impurities in each separated ( n , m ) species were metallic nanotubes and other semiconducting chiralities. The absence of metallic peaks in the optical absorption spectra of the S-SWCNT fractions ( Fig. 4a ) indicates that these ( n , m ) fractions exhibited high electronic purities. Raman spectroscopy ( Supplementary Fig. S6 ) also confirmed the high electronic purity of the ( n , m ) fractions. Metallic peaks were not observed for any of the ( n , m ) fractions. Therefore, the risk of metallic impurity can be ignored when calculating the purities of the separated ( n , m ) fractions. In addition, the low relative intensities of the D bands (near 1,300 cm −1 ) in the Raman spectra suggest that the nanotubes separated by SS-MUGEC contained few defects. We used the method described in ref. 15 ( Supplementary Figs S7 and S8 ) to estimate the chirality enrichment of each ( n , m ) fraction; the results are given in Table 1 . The ( n , m ) purities are comparable with those recently obtained by the DNA wrapping method [20] . We also measured the fluorescence intensity of each ( n , m ) fraction as a function of the excitation and emission wavelengths ( Fig. 4c ). The resulting contour plots further confirmed the significant enrichment of the single-chirality species. Table 1 The purity and product yield of each ( n , m ) enriched semiconducting species. Full size table A high yield is important for an effective sorting method. To assess the purification yield of each ( n , m ) fraction after the second separation by the SS-MUGEC method, we converted the absorption spectrum intensity of each ( n , m ) nanotube fraction into an SWCNT mass concentration [30] . The yields of purified ( n , m ) nanotubes were estimated using the ratios of the amounts of collected purified ( n , m ) fractions to those of the corresponding ( n , m ) nanotubes in the HiPco SWCNTs that were initially loaded. The results are given in Table 1 , indicating high purification yields. In Figure 4 and Table 1 , only the ( n , m ) fractions with the highest purities are presented. A few fractions that sorted in different columns and collected in the second separation contained substantial amounts of the ( n , m ) species, with varying degrees of purity ( Supplementary Fig. S9 ). Accordingly, the purification yield of a specific ( n , m ) nanotube depends on the degree of purification. Because of the repeatable nature of the SS-MUGEC method, low-purity ( n , m ) fractions can be collected for reseparation to improve their chirality purity, and we expect that it will be possible to completely separate each ( n , m ) fraction from the mixture after several rounds of separation. Note that increasing the purification times influences the final purification yield and increases the cost because irreversible adsorption and column degradation is a ubiquitous problem in liquid chromatography, although here less than 1wt % of the nanotubes were irreversibly adsorbed on the gel columns in each separation run. The purification yield and efficiency of a specific ( n , m ) can be improved markedly if it is present at a high level in the starting material (for example, (6, 5)-enriched Comocat nanotubes [31] ). We also attempted to perform chirality separation of arc plasma jet-grown SWCNTs with diameters of 1.28–1.52 nm [32] . The results indicated that the chirality separation of nanotubes with diameters larger than 1.4 nm was not observed using the SS-MUGEC method and the present separation parameters. To clarify the order-dependent chirality separation mechanism, we characterized the morphologies of the separated ( n , m ) nanotubes using atomic force microscopy (AFM). The AFM images indicated little difference in length among the different ( n, m ) nanotubes ( Supplementary Fig. S10 ), suggesting that a length difference of the nanotubes was not the main reason for their chirality separation. Note that the S-SWCNTs trapped on an allyl dextran-based size-exclusion gel can be easily desorbed and eluted by injecting high-concentration surfactant (SDS). This result suggests that an SDS coating fully covering the nanotubes minimizes their interactions (such as van der Waals or hydrophobic) with the gel. The order-dependent chirality separation is thought to originate from different degrees of SDS coating coverage on the nanotube surfaces, which scales the interaction strength of each ( n , m ) single-chirality nanotube with the gel. The morphology and coverage of SDS coatings on nanotubes have recently been reported to be dependent on nanotube structure [33] , [34] . To address this issue, we analysed the relationships between the separation order of ( n , m ) nanotubes and their chiral angle ( θ ), diameter ( D t ) and smallest bond curvature radius ( R c , R c = D t /(2 cos 2 ) (30− θ )) [12] , [35] . 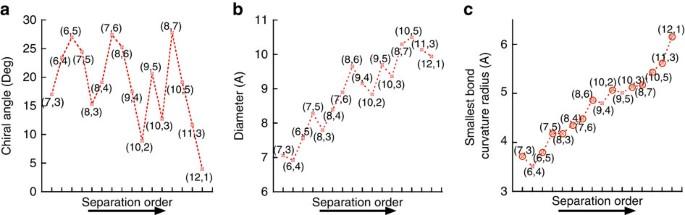Figure 5: The relationship between the separation order of (n,m) nanotubes and their physical structures. (a) Chiral angle. (b) Diameter. (c) Smallest bond curvature radius. The separation orders for the (9, 5), (10, 5) and (11, 3) nanotubes were determined in the first separation process. (c) Indicates that the separation order of (n,m) semiconducting species depends most strongly on their smallest C–C bond curvature radius (that is, their largest bond curvature). As presented in Figure 5 , the relationship between the smallest bond curvature radius of the ( n , m ) nanotubes and the separation order displays a relatively smooth increasing tendency compared with the relationships between separation order and chiral angle or diameter, indicating that the nanotubes that interact more strongly with the gel basically have smaller bond curvature radii, except for (6, 4), (9, 4) and (9, 5). We believe that differences in the surface π-electron states of the various S-SWCNTs resulting from differing bond curvatures affect the interaction between S-SWCNTs and SDS and cause the variation in the SDS coating coverage. Therefore, this method for the chirality separation of nanotubes depends strongly on their curvature. SWCNTs with diameters larger than 1.4 nm generally have a larger bond curvature radius and hence a higher SDS coating coverage, leading to weak interaction with the gel and therefore low-resolution chirality separation or no separation. Metallic nanotubes are generally thought to be fully covered by SDS [22] , and they have a much weaker interaction with the gel than do semiconducting nanotubes. The full SDS coating coverage on metallic nanotubes is attributed to their different electronic structures from semiconducting nanotubes, resulting in a strong interaction with the SDS surfactant. Accordingly, the metallic nanotubes were collected as unbound nanotubes and are difficult to separate with the present method. Figure 5: The relationship between the separation order of ( n , m ) nanotubes and their physical structures. ( a ) Chiral angle. ( b ) Diameter. ( c ) Smallest bond curvature radius. The separation orders for the (9, 5), (10, 5) and (11, 3) nanotubes were determined in the first separation process. ( c ) Indicates that the separation order of ( n , m ) semiconducting species depends most strongly on their smallest C–C bond curvature radius (that is, their largest bond curvature). Full size image In summary, the new phenomenon of a structure-dependent interaction strength of SWCNTs with an allyl dextran-based size-exclusion gel was observed. This interaction permitted nanotubes to be separated on the basis of their chirality. On the basis of these results, we developed a highly effective SS-MUGEC method for large-scale chirality separation of SWCNTs that can be used for the simultaneous separation of M- and S-SWCNTs. One of the most attractive features of this method is that the separation process uses only a single surfactant, therefore the separation of SWCNTs can easily be repeated to improve the chirality purity level following a simple dilution of the SDS solution. After two separations of HiPco SWCNTs, we were able to purify at least 13 highly enriched ( n , m ) S-SWCNT species. More importantly, the SS-MUGEC method is simple, rapid and inexpensive. This method realizes the chirality separation of SWCNTs on a large scale, and we expect to be able to produce single crystals of single-chirality nanotubes in the near future. We believe that this separation method will open up a new research field and accelerate the use of SWCNTs in practical applications. Dispersion of SWCNTs Single-wall carbon nanotubes produced by high-pressure catalytic CO (HiPco) decomposition (HiPco, RØ500, 1.0±0.3 nm) were purchased from Carbon Nanotechnologies Inc. and were used as the starting material for the nanotube separation trials. Aliquots of 100 mg of HiPco SWCNTs were dispersed in 100 ml of purified water with 2 wt% SDS (99%, Sigma-Aldrich) using an ultrasonic homogenizer (Sonifire 450D, Branson) equipped with a 0.5-inch. flat tip for 20 h at a power density of 20 W cm −2 . To prevent heating during sonication, the bottle containing the sample solution was immersed in a bath of cold water. To remove the residue of catalytic metal particles, nanotube bundles and impurities, the dispersed sample solution was centrifuged at 197,000 g for 15 min in a swinging-bucket rotor (S52ST, Hitachi Koki). The upper 90% of the supernatant was collected and used for gel chromatography. Overloading effect Medical plastic syringes (10 ml; 8 cm in length and 1.5 cm in inner diameter) were used as the columns. Allyl dextran-based size-exclusion gels (Sephacryl gel, S-200 HR or S-300 HR, GE Healthcare) were used as the gel media. Two gel columns were prepared by filling the same amount of allyl dextran-based size-exclusion gel (1.4 ml of gel beads) into two syringes that were labelled Col. 1 and Col. 2 ( Fig. 1a ). Before filling with gel beads, the outlet of each syringe was plugged with cotton. After the gel columns were equilibrated with a 2 wt% SDS solution, 1- and 8-ml aliquots of the SWCNT dispersion were applied to Col. 1 and Col. 2, respectively. Next, a 2 wt% aqueous SDS solution was used to elute the unbound nanotubes until no nanotubes were detected in the eluent. The nanotubes adsorbed on the two gel columns were desorbed and collected by injection with a 5 wt% SDS solution. A video of the separation process was recorded (see Supplementary Movie 1 ). The nanotubes adsorbed by each of the two columns were characterized using optical absorption spectra ( Fig. 1d ) and PL contours (see Supplementary Fig. S1 ). Chirality separation by multicolumn gel chromatography Chirality separation was performed using a SS-MUGEC method. In this method, several 10-ml syringes filled with 1.4 ml of allyl dextran-based size-exclusion gel beads (Sephacryl S-200 HR or S-300 HR, GE Healthcare) were connected vertically in series. The top of each column was open, and there were no seals between the stacked columns. A schematic diagram of the SWCNT separation process is presented in Figure 2a and Supplementary Figure S2 . After the gel columns were equilibrated with a 2 wt% SDS solution, a 5–10 ml aliquot of the SWCNT dispersion was applied onto the top column. Subsequently, a 2 wt% SDS aqueous solution was added onto the top column to elute the unbound nanotubes. The unbound SWCNTs flowed from one column to another by gravity and were finally collected from the bottom column. The trapped semiconducting nanotubes were desorbed and collected from each column by disconnecting the gel column series and adding a 5 wt% SDS aqueous solution to each column. After equilibrating the gel columns with 2 wt% aqueous SDS, we repeated the above procedure by loading the unbound SWCNTs until no semiconducting SWCNTs were trapped in the gel columns. The remaining unbound nanotubes were identified as highly metal-enriched nanotubes. The semiconducting nanotubes collected from each column were confirmed to be separated by diameter and chirality ( Fig. 2 , Supplementary Figs S3 and S4 ). Single-chirality separation Single-chirality separation from each semiconducting nanotube fraction was performed using the SS-MUGEC method. Several 10-ml medical syringes, as described above, were connected vertically in series. Before separation, the SDS concentration in each semiconducting nanotube fraction was diluted to 2 wt%. After the gel columns were equilibrated with 2 wt% SDS solution, the diluted semiconducting fractions (5–10 ml, 16 μg ml −1 ) were applied to the top column, and a 2 wt% SDS aqueous solution was then added to the series of columns to elute the unbound nanotubes. The semiconducting nanotubes adsorbed in each column were collected by injecting a 5 wt% SDS solution. The second separated semiconducting nanotube fractions were characterized by optical adsorption spectra and PL contours ( Figs 3 and 4 ; Supplementary Fig. S5 ), which confirmed that at least 13 different ( n , m ) species were isolated from the HiPco-grown SWCNTs. Optical absorption measurement Optical absorption data were recorded from 200 to 1,350 nm with an UV−vis−NIR spectrophotometer (SHIMADZU SolidSpec−3700DUV), using a quartz cell with a path length of 5 mm. Pristine HiPco SWCNTs and sorted samples were dispersed in 5 wt% aqueous SDS solution. The spectral resolution was 1 nm. For the HiPco SWCNTs, the absorption peaks at 850−1,350, 500−850, 330−450 and 300−400 nm were derived from the first (S 11 ), second (S 22 ), third (S 33 ) and fourth (S 44 ) optical transitions of the semiconducting SWCNTs, respectively ( Supplementary Fig. S5 ) [2] . The absorbance peak at 400−650 nm represented the first optical transition of metallic (M-) SWCNTs (M 11 ) [2] . The absorption peaks observed in the shorter wavelength region (200–300 nm) indicate the UV optical absorption characteristic of the nanotubes. Raman spectra measurements Raman spectra were measured in aqueous SDS solution at a concentration of 5 wt% using a triple monochromator (Bunkou-Keiki, M331-TP) equipped with a charge-coupled device detector. The samples were excited at excitation wavelengths of 633, 561 and 514 nm using a power of 10 mW. Photoluminescence spectra measurements We measured near-infrared fluorescence intensity as a function of excitation and emission wavelengths for pristine HiPco and sorted HiPco samples in aqueous SDS solution (concentration 5 wt%) with a spectrofluorometer (HORIBA, NanoLog) equipped with a liquid-nitrogen-cooled InGaAs near-IR array detector. The excitation wavelength was varied from 450 to 850 nm in 5-nm steps, and the emission wavelength was varied from 850 to 1,400 nm in 5-nm steps. The spectral slit widths were 7 nm for both excitation and emission. The raw data were corrected with instrumental factors. AFM observation Atomic force microscopy was used to observe the morphologies of the sorted nanotubes. The samples for AFM characterization were prepared by casting an SWCNT dispersion onto an SiO 2 /Si substrate coated with a self-assembled monolayer of 3-aminopropyltriethoxysilane (Sigma-Aldrich) and further rinsing it with water. After drying the sample with a stream of dry N 2 gas, AFM images were recorded using a dynamic force mode AFM (SII, SPI3800) at a resolution of 512 samples per line. Purity evaluation of sorted SWCNTs PeakFit software was used to simulate the near-infrared spectra as sums of Voigt functions representing individual ( n , m ) species with peaks from 800 to 1,350 nm. The purity of each ( n , m ) fraction was computed as the ratio of the area of the dominant peak to the sum of the areas of all peaks. Assessment of purification yield for ( n, m ) tubes The yield of purified ( n , m ) fractions was estimated as the ratio of the amount of the collected purified ( n , m ) fractions to that of the corresponding ( n , m ) nanotubes in the initially loaded HiPco SWCNTs. The amount of each ( n , m ) fraction was evaluated by converting its absorption spectrum intensity into a mass concentration [30] . How to cite this article: Liu, H. et al . Large-scale single-chirality separation of single-wall carbon nanotubes by simple gel chromatography. Nat. Commun. 2:309 doi: 10.1038/ncomms1313 (2011).